Transmission-blocking interventions eliminate malaria from laboratory populations Transmission-blocking interventions aim to reduce the prevalence of infection in endemic communities by targeting Plasmodium within the insect host. Although many studies have reported the successful reduction of infection in the mosquito vector, direct evidence that there is an onward reduction in infection in the vertebrate host is lacking. Here we report the first experiments using a population, transmission-based study of Plasmodium berghei in Anopheles stephensi to assess the impact of a transmission-blocking drug upon both insect and host populations over multiple transmission cycles. We demonstrate that the selected transmission-blocking intervention, which inhibits transmission from vertebrate to insect by only 32%, reduces the basic reproduction number of the parasite by 20%, and in our model system can eliminate Plasmodium from mosquito and mouse populations at low transmission intensities. These findings clearly demonstrate that use of transmission-blocking interventions alone can eliminate Plasmodium from a vertebrate population, and have significant implications for the future design and implementation of transmission-blocking interventions within the field. Malaria is a global disease of man caused by parasites of the genus Plasmodium , which are transmitted exclusively by Anopheles mosquitoes. There are an estimated 219 million human malaria cases annually—90% of resulting deaths occur in Africa, with children under the age of 5 and pregnant women most severely affected [1] . If we are to contemplate control or elimination of malaria, it is now recognized that we must attack Plasmodium directly on two fronts; we must reduce the impact of disease upon the infected individual, and at the population level we must reduce the number of new infections. Current analyses suggest that to reduce new infections, potentially the most effective point to attack the parasite is during its transmission through the mosquito vector [2] , a process that in the field, commonly results in infection of <5 parasites per mosquito [3] , [4] . Targeting Plasmodium within the vector (using either transmission-blocking drugs or vaccines) aims to reduce both the prevalence of infected mosquitoes and the parasite burden in individual infected insects, consequently reducing the exposure of a human population to potentially infectious mosquitoes. Successful use of an anti-malarial transmission-blocking intervention (TBI) should, as its overall objective, aim to reduce the number of secondary malarial infections. This important parameter has never been experimentally investigated. Malaria endemicity is typically measured using the entomological inoculation rate (EIR). It is calculated by multiplying the host biting rate (the average number of bites per person per unit time) by the sporozoite rate (the proportion of biting mosquitoes which contain salivary gland sporozoites). Mathematical modelling studies have indicated that TBIs could be most effective in areas of low transmission with low EIRs [5] , [6] . Other studies have questioned whether usage of TBIs could reduce malaria infection and malaria-related morbidity and mortality across all transmission settings [7] . To our knowledge, laboratory-based evidence to support these in silico predictions does not exist. Given the current international interest in interrupting malaria transmission, a wide range of novel TBIs have been investigated using a variety of assays designed to measure efficacy. These assays (for example, the standard membrane feeding assay (SMFA) and direct feeding assay (DFA)), typically measure parasite development within the mosquito, assessing efficacy as reduction in parasite prevalence or intensity [8] , [9] . Although undeniably informative, such assays have highly variable (and density-dependent) readouts [10] . Moreover, the assay end points do not measure reduction in the number of secondary malarial infections, thus preventing the determination of transmission reductions required to have a significant impact in different endemic situations. Future regulatory approval for TBIs may require laboratory data demonstrating the effectiveness of these interventions: currently, no such data have been published. Current go/no-go efficacy thresholds for an effective transmission-blocking vaccine have been suggested to be an 80% reduction in oocyst intensity in the mosquito midgut [11] , [12] . However, we have no practical evidence whether, and under what field conditions (for example, transmission intensities/EIR), such levels of inhibition could effectively reduce transmission. Here we report a transmission-based population ‘bottle’ study to assess how a TBI will reduce the number of secondary cases of malarial infection if applied over multiple transmission cycles within closed populations of insect and vertebrate hosts. We have used the rodent malaria parasite P. berghei , the only mammalian system in which these experiments are at present both technically and ethically possible. The impact of a TBI is investigated at five different transmission intensities, which are generated by altering the number of (potentially) infectious mosquitoes that bite individual naive mice (that is, one, two, three, four or five bites per mouse)—which we term the mosquito biting rate (MBR). Using a previously characterized TBI, atovaquone (ATV) [13] , we have shown that a TBI that only partially reduces oocyst intensity and prevalence can, in the absence of any other intervention, eliminate Plasmodium infection from both mosquito and mouse populations within three cycles of transmission at low MBRs. At higher MBRs, the parasite is not eliminated from either population. This is the first practical demonstration that successive rounds of anti-parasite transmission blockade have the potential to eliminate malarial infection in a mammalian population. We extend the impact of our findings to inform the potential applications of TBI usage on a global scale, and suggest that a significant fraction of malaria affected communities could benefit from the application of TBIs of a similar or higher efficacy. Assessment of intervention efficacy by DFA To establish the effect of transmission blockade on parasite dynamics over successive rounds of transmission, we used the proven and highly reproducible transmission-blocking drug ATV. ATV is a broad range 8-aminoquinoline anti-malarial, with well-established activity against transmission stages [13] . Transmission-blocking (TB) efficacy, as classically defined at the chosen dose (0.5 μg kg −1 , intraperitoneal (i.p. )), was determined using the standard DFA [14] ( Fig. 1 ). The drug achieved a mean 57.3% reduction in oocyst intensity (95% confidence interval (CI) 38.9–70.2%) and a 32.3% reduction in infection prevalence (95% CI 11.1%–47.6%) (hear after referred to as an efficacy of TB ooc 57/32%). Negative controls received dimethyl sulfoxide (DMSO) (i.p.). 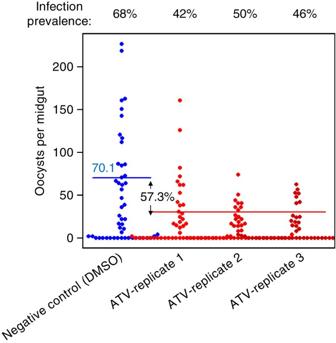Figure 1: Transmission-blocking impact of atovaquone onP. bergheias determined by direct-feed assay. ATV dosage used was 0.5 μg kg−1. An equal volume of DMSO (i.p.) was used as a negative control. Oocysts present on the mosquito midguts were counted 10 days post feeding. Each data point represents a single mosquito within an individual treatment group.X-axis points represent individual mice. Blue horizontal line indicates the mean number of oocysts for the negative control treatment; red horizontal line indicates the mean number of oocysts for all three ATV replicates. Mean ATV impact from three replicates was 57.3% reduction in oocyst intensity and a 32.3% reduction in infection prevalence (hereafter referred to as TBooc57/32%). Figure 1: Transmission-blocking impact of atovaquone on P. berghei as determined by direct-feed assay. ATV dosage used was 0.5 μg kg −1 . An equal volume of DMSO (i.p.) was used as a negative control. Oocysts present on the mosquito midguts were counted 10 days post feeding. Each data point represents a single mosquito within an individual treatment group. X -axis points represent individual mice. Blue horizontal line indicates the mean number of oocysts for the negative control treatment; red horizontal line indicates the mean number of oocysts for all three ATV replicates. Mean ATV impact from three replicates was 57.3% reduction in oocyst intensity and a 32.3% reduction in infection prevalence (hereafter referred to as TB ooc 57/32%). Full size image Experimental design of transmission-based population model Five successive rounds of mouse–mosquito–mouse transmission were performed ( Fig. 2 , Supplementary Data S1 ). Five paired experiments were conducted in parallel, at five different MBRs. Individual naive mice were exposed to given numbers (1–5) of potentially infectious mosquitoes taken at random from a larger population of Anopheles stephensi . Within individual paired experiments, one population was exposed to the TBI and one was maintained without TBI treatment. To ensure comparability of data, all populations were seeded from the same mosquito and parasite populations. For every cycle, parasite transmission was monitored by measuring the following outputs: parasitemia/gametocytemia in mice from the initial population, oocyst intensity/prevalence (and related TB impact), proportion of biting mosquitoes with salivary gland sporozoites and prevalence of blood-stage infection in subsequent mouse populations. 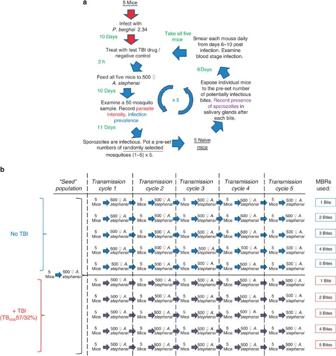Figure 2: Experimental design of population transmission experiments. (a) A single experimental round of mouse–mosquito–mouse transmission usingP. bergheiandAnopheles stephensi. (b) Schematic of performed population transmission experiments. Total number of mosquitoes and mice used are described. Ten paired parallel transmission experiments were performed, for five successive cycles of transmission. Red arrows indicate transmission carried out in presence of TBI (TBooc57/32%), blue arrows indicate transmission carried out in absence of TBI (with control). Five MBRs of one to five (potentially infected mosquito bites per naive mouse) were examined. Figure 2: Experimental design of population transmission experiments. ( a ) A single experimental round of mouse–mosquito–mouse transmission using P. berghei and Anopheles stephensi . ( b ) Schematic of performed population transmission experiments. Total number of mosquitoes and mice used are described. Ten paired parallel transmission experiments were performed, for five successive cycles of transmission. Red arrows indicate transmission carried out in presence of TBI (TB ooc 57/32%), blue arrows indicate transmission carried out in absence of TBI (with control). Five MBRs of one to five (potentially infected mosquito bites per naive mouse) were examined. Full size image Effect of intervention on transmission at different biting rates In these studies, we have expressed the impact of the TBI on successive rounds of transmission as the effect on the parasite within the mosquito vector (assessed as infection prevalence and intensity), or within the vertebrate host (assessed as prevalence of blood-stage infection at day 10 post bite) ( Fig. 3 ). 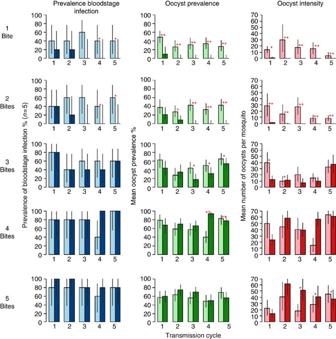Figure 3: Effect of a TBI with an efficacy of TBooc57/32% on host/vector infection over successive rounds of transmission. Each row shows a different MBR with mice receiving either one, two, three, four or five bites per generation. The first column (blue bars) shows the number of mice developing parasitemias over the different rounds of the experiment, the second column (green bars) the percentage of mosquitoes developing oocysts and third column (red bars) the mean intensity of oocyst per mosquito. Lighter bars denote control group with no intervention while darker bars signify those administered with the TBI. Vertical grey lines indicate 95% CIs. Red stars indicate the number of rounds required for there to be a statistically significant difference between the control and treatment arms of the experiment (*P<0.05, **P<0.001). At each generation at a single biting rate, for micen=10, mosquitoesn=1,000. Figure 3: Effect of a TBI with an efficacy of TB ooc 57/32% on host/vector infection over successive rounds of transmission. Each row shows a different MBR with mice receiving either one, two, three, four or five bites per generation. The first column (blue bars) shows the number of mice developing parasitemias over the different rounds of the experiment, the second column (green bars) the percentage of mosquitoes developing oocysts and third column (red bars) the mean intensity of oocyst per mosquito. Lighter bars denote control group with no intervention while darker bars signify those administered with the TBI. Vertical grey lines indicate 95% CIs. Red stars indicate the number of rounds required for there to be a statistically significant difference between the control and treatment arms of the experiment (* P <0.05, ** P <0.001). At each generation at a single biting rate, for mice n =10, mosquitoes n =1,000. Full size image In the absence of TBI, at any chosen MBR, parasite transmission is broadly stable across five successive cycles, with no significant change in oocyst intensity/prevalence in the mosquito population, or prevalence of blood-stage infection in the vertebrate population. As expected, increasing the MBR increased the proportion of mice infected. Following administration of the TBI, at lower MBRs (one and two bites), Plasmodium was progressively reduced in terms of oocyst intensity and prevalence (in the mosquito population), as was blood-stage parasitemia (in the vertebrate population). The parasite was subsequently eliminated. At an MBR of 1, the parasite is eliminated from the mosquito population by cycle 2, and from the mouse population by cycle 3. At an MBR of 2, elimination from both mosquito and mouse population occurs by cycle 3. At MBRs of 3 or higher, the parasite is not eliminated from the mosquito population and there is no significant reduction observed in the prevalence of blood-stage infection within the vertebrate hosts. The overall effectiveness of an intervention can be quantified by estimating its ability to reduce the basic reproduction number (that is, R 0 ), the average number of secondary cases of malaria resulting from a single case in an otherwise uninfected population. Correspondingly, the term R C is often used to describe the basic reproduction number under control interventions. If R C is sustainably reduced to <1, malarial transmission is considered non-sustainable. The magnitude of the reduction in R 0 or R C has been termed the ‘effect size’ [15] and measures the ability of an intervention to reduce the probability of transmission from human-to-vector and vector-to-human. If it is assumed that that all infectious mosquitoes are equally infectious then the effect size can be estimated by fitting a chain binomial model to the data [16] . Overall, our experiment indicates that use of our TBI (with TB ooc 57/32%) over successive transmission cycles results in an effect size of 20.4% (95% CI 15.2–24.9%). Further data concerning oocyst intensity, oocyst prevalence and proportion of biting mosquitoes with salivary gland sporozoites over successive rounds of transmission are provided in Supplementary Table S1 . To preclude the possibility of drug resistance having emerged at the higher transmission intensities after repeated rounds of ATV treatment, at the end of five transmission cycles, surviving parasites (from experiments conducted at transmission intensities ≥3) that had been exposed to drug were tested for ATV resistance. All parasites demonstrated ATV sensitivity identical to the originating wild-type parasite ( Supplementary Fig. S2 ). Anti-malarial TBIs aim to interrupt the development of the parasite through the mosquito host, and therefore reduce the number of secondary malarial infections within a human population. The potential effectiveness of any TBI under field conditions will depend on a number of highly variable factors, including endemic transmission/EIR levels, TBI efficacy, TBI coverage levels, the distribution of the number of oocysts per mosquito and the proportion of biting mosquitoes that carry sporozoites [12] . Currently, assays to determine TBI effectiveness do not measure the reduction in the number of secondary malarial infections, but typically measure intermediate parasite outputs within the insect vector [8] , [10] , [17] . As a result, there are no primary data to link the required TBI efficacy to reduction in secondary infection within the coindigenous human population. We report the first proof of concept studies to link these two end points, and further demonstrate the critical importance of understanding their dependence upon transmission intensity. This study further outlines the importance of multigenerational transmission studies when assessing the impact of a TBI. Traditionally, TBI impact is measured within one transmission step (host-to-vector). Current TBI development pipelines suggest that an 80% reduction in oocyst intensity [11] , [12] should be a threshold efficacy for future development. We show that both of these conventions fail to appreciate that a TBI of incomplete efficacy (here TB ooc 57/32%) can eliminate Plasmodium from both mosquito and vertebrate populations at low transmission levels over successive rounds of application. This has obvious implications for the future design and usage of TBIs in highly variable endemic situations. We are not suggesting using ATV as part of a malaria control programme, or utilizing a TBI of this efficacy in the field; however, we can certainly expect that the (modest) efficacy examined here will be exceeded by that of TBIs currently under development, for example, SMFA data using anti-Pfs25 antibodies have resulted in up to a 96% reduction in oocyst intensity [18] , [19] , [20] , and anti-Pfs48/45 and Pfs230 antibodies have reported up to 90% and 100% reductions in intensity, respectively [21] , [22] , [23] . Lead candidates for development as transmission-blocking drugs also demonstrate significantly higher potency, for example, the spiroindolone drug NITD609 has demonstrated a dose-dependent effect on P. falciparum oocyst counts in the SMFA, with a TB ooc of 100/100% observed at 500 nM ( [24] ). This study provides clear evidence that the ability of a TBI to eliminate malaria will depend on the transmission intensity. Transmission was halted in populations where each mouse received one or two bites and was maintained in those receiving three, four or five bites. A significant reduction in mosquito infection (both oocyst prevalence and intensity) was observed in the group which received three bites with application of TBI. This may subsequently result in fewer vertebrate infections, although as only five mice were used in each population it was not possible to show a statistically significant reduction at this MBR. Previously, theoretical studies to examine malarial transmission have predicted that TBIs could impact the number of malarial cases within the field under a variety of conditions, particularly at levels of low transmission [5] , [6] . Other studies have additionally suggested that use of a TBI at relatively low effective coverages could give a substantial reduction in the number of malarial cases [25] . Our simple lab-based, multi-cycle population model supports both of these conclusions, indicating that usage of a TBI with a modest efficacy will achieve elimination of Plasmodium berghei within the laboratory at levels of transmission where MBR ≤2. Further application of these experiments must examine the required efficacies and coverages for TBIs to eliminate Plasmodium at higher host biting rates, such that we will be able to provide experimental justification of the TB ooc efficacy required for TBIs to achieve elimination in different transmission settings. We are acutely aware that the transmission intensities described within this study may not be directly translatable to transmission as measured in natural populations of human malaria. Experimental studies have determined that vertebrate–mosquito–vertebrate transmission is much more efficient in our laboratory model than in naturally found parasite–vector combinations [4] , [9] . Nevertheless, if a TBI candidate had an effect size in humans of 20.4%, as was seen here within our rodent model system, then epidemiological theory indicates that if it was given and maintained in 100% of the population it would result in malarial elimination in areas where the R c was <1.255. Recent disease maps [26] illustrate that 74.77% of the malaria affected population and 63.14% of malaria affected areas are located in areas where an R c <1.255 ( Fig. 4 ). These combined data suggest that widespread use of a TB vaccine or drug with a higher efficacy (for example, those examined in [17] , [18] , [19] , [20] , [21] , [22] , [23] ) could have significant and widespread implications for global health and malarial burden. 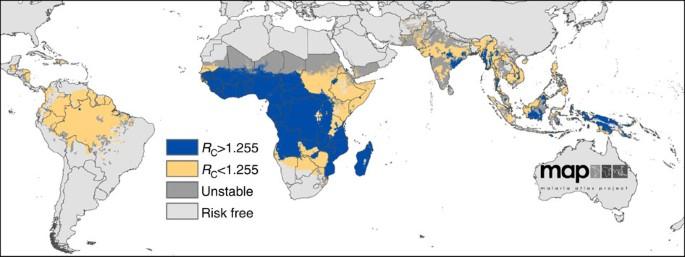Figure 4: Spatial global malaria distribution of areas withRc<1.255. Blue:Rc>1.255, yellow:Rc<1.255. Areas of unstable transmission (medium grey areas) or no risk (light grey) are also indicated. Figure 4: Spatial global malaria distribution of areas with R c <1.255. Blue: R c >1.255, yellow: R c <1.255. Areas of unstable transmission (medium grey areas) or no risk (light grey) are also indicated. Full size image The wide range of new TBIs (both drugs and vaccines) currently under development will require Phase 3, likely to be placebo controlled, randomized trials where the unit of randomization will be a village and the outcome will be the reduction in transmission as measured by decreased incidence of infection [12] . Recognizing the high financial cost of these studies, it is important to develop realistic go/no-go criteria for efficacy before progressing TBI development to this level. The studies described here may offer a robust, accurate, safe and cost-effective manner to experimentally examine these critical parameters. The strength of the experimental design we have developed is that our protocol provides a technically accessible and ethical framework to examine, over multiple cycles of transmission, the population dynamics of transmission blockade in a host population, with direct control of individual regulating parameters (for example, TBI efficacy) which in the field may be simultaneously uncontrollable, variable and often unmeasurable. Our data and subsequent analyses strongly support the notion expressed in numerous other studies [5] , [12] , [27] , [28] that malaria control presents variable challenges across its transmission spectrum, and that strategic planning for control or elimination should consider a number of factors, with particular emphasis on the efficacy of TBI required, and the transmission intensity/EIR in the targeted area. The design and field implementation of an anti-malarial TBI is likely to be both complex and multifaceted, although our data suggest that we may be closer than we previously thought to the utilization of an effective anti-malarial TBI. DFA to establish ATV efficacy Six days before mosquito feed, 4- to 10-week-old female TO mice were treated i.p. with 200 μl phenylhydrazine (6 mg ml −1 in PBS; ProLabo, UK). Three days before feeding, mice were infected i.p. with 10 7 –10 8 parasitized red blood cells, infected with P. berghei ANKA 2.34. One day before feeding, mosquitoes were placed in an appropriate container and starved for 24 h. For each mouse, ~60 female A. stephensi (SD 500) mosquitoes were potted. On the day of the mosquito feed, parasitemia, gametocytemia and presence of exflagellation were recorded as described previously [14] . Mice were injected i.p. with ATV (Sigma Aldrich, no. A7968) dissolved in DMSO to give a final dose of 0.5 μg kg −1 in 100 μl volume. Hundred microlitres DMSO alone (i.p.) was used as negative control. Post treatment, mice were left for 2 h, after which, mice were anesthetized and pots of starved A. stephensi mosquitoes were allowed to feed on each infected mouse. Twenty four hours after feeding, mosquitoes were briefly anesthetized with CO 2 , and unfed mosquitoes were removed. Mosquitoes were maintained on 8% (w/v) fructose, 0.05% (w/v) p-aminobenzoic acid at 19 °C and 80% relative humidity. At day 10 post feeding, 50 mosquito midguts were dissected, and oocyst prevalence and intensity recorded. For inhibition calculations these values were compared with mean oocyst intensity and infection prevalence in control (DMSO) groups. All care and handling of animals was in accordance with the Guidelines for Animal Care and Use prepared by Imperial College London. The efficacy of the intervention was calculated (over all replicate experiments) using a generalized linear mixed effects model [10] . Treatment was included as the fixed effect while efficacy between replicates was allowed to vary at random between replicates. A binomial error structure was used for the parasite presence/absence data while a zero-inflated negative binomial distribution was used to describe mosquito oocyst intensity. Efficacy 95% CI estimates were generated by bootstrapping methodology (with 100,000 replicates). Successive rounds of P. berghei transmission Five successive rounds of mouse–mosquito–mouse transmission were performed, with general parasite maintenance carried out as described [12] . Briefly, for each individual transmission setting under investigation, two groups of five P. berghei ANKA 2.34 parasites were maintained in 4- to 10-week-old female TO mice by syringe inoculation (i.p. ), followed by mouse–mosquito–mouse passage. For each transmission cycle infections were monitored on Giemsa-stained tail blood smears as described [14] . At day 10 post infection, individual groups of mice were treated with either ATV at a final dose of 0.5 μg kg −1 in 100 μl volume (i.p. ), or 100 μl DMSO alone (i.p.) as negative control. Post treatment, mice were left for 2 h, after which, groups of five mice were anesthetized and exposed to cages containing 500 starved female A. stephensi (SD 500) mosquitoes. Unfeds were removed and mosquitoes were maintained as described above. On day 10 post feeding, from a 50-mosquito sample taken from each individual cage, midguts were dissected, and oocyst prevalence and intensity recorded. For each mosquito population, oocyst numbers were counted and mean oocyst intensity was calculated. To calculate inhibition, this number was compared with the relevant control group. Remaining mosquitoes were maintained until 21 days post infection, when salivary gland sporozoites were at their peak [14] . Individual transmission intensities were established by exposing individual, anesthetized naive mice to set numbers (between 1 and 5) of potentially infectious mosquitoes, selected at random from the larger population. Successful feeding was confirmed by the presence of blood in the abdomen of mosquitoes after 20 min. Post feeding, individual mosquitoes were dissected to determine the percentage with salivary gland sporozoites, and salivary gland sporozoites scored on a log scale (score of 0=no sporozoites visible; 1=1–10 sporozoites visible; 2=10–100 sporozoites visible; 3=100–1,000 sporozoites visible; 4=1,000+ sporozoites visible). Post feeding, mice were maintained for 10 days. From days 6 to 10, naive mice were smeared daily as described in [14] . At day 10 post infection, P. berghei gametocytes present in infected mice are at their optimal infectivity to mosquitoes [29] . At this time, groups of mice were treated with either ATV at a final dose of 0.5 μg kg −1 (i.p. ), or DMSO alone (i.p.). Post treatment, mice were left for 2 h, after which, groups of five mice were anesthetized and exposed to new cages containing 500 naive starved female A. stephensi (SD 500) mosquitoes, completing a cycle of mouse–mosquito–mouse transmission. For each individual experiment, five successive rounds of transmission were performed. 10 individual experiments were performed in parallel, at five different levels of transmission intensity (1, 2, 3, 4 and 5 mosquitoes exposed to naive mice). Five experiments were performed with ATV (0.5 μg kg −1 ), and five paired populations with DMSO alone. After five rounds of cyclic transmission, from each experiment, P. berghei -infected blood was collected by cardiac puncture, and tested for persisting sensitivity to ATV by DFA as described above. Results demonstrating continued drug sensitivity are shown in Supplementary Fig. S2 . Data regarding proportion of biting mosquitoes with salivary gland sporozoites, oocyst intensity and oocyst prevalence from all experiments over five successive rounds of transmission are included in Supplementary Data . Data regarding the proportion of biting mosquitoes with salivary gland sporozoites over successive rounds of transmission is provided in Supplementary Table S1 , and data regarding continued sensitivity of P. berghei after five cycles of transmission is provided in Supplementary Fig. S2 . Statistical analysis of cyclic transmission Generalized linear models were used to determine whether administering a TBI significantly influenced mouse and mosquito infectivity over the different rounds of infection for a population with a specific biting rate. For each biting rate, the model determined the number of rounds of the life cycle required before including information on whether the mosquito/mouse was in the control or intervention arm significantly improves the fit of the model (using a likelihood ratio test). A binomial error structure was used for the parasite presence/absence data while a zero-inflated negative binomial distribution was used to describe mosquito oocyst intensity. Ninety-five per cent CIs were generated using bootstrapping methodologies (with 100,000 replicates). Calculation of effect size of intervention Let p i denote the prevalence of infection in mice and q i the prevalence in mosquitoes at generation i (when i =0..5). Generation 0 is initiated in mice with p 0 =1. Let r denote the (per bite) probability of infection from an infected mosquito to a susceptible mouse, s the probability of infection from an infected mouse to a susceptible mosquito and m the MBR. Assuming that the probability that a mosquito transmits the infection is the same, irrespective of the number of bites the mouse receives, then the probability that a susceptible mouse is infected after exposure to m mosquito bites in generation i is described in equation (1): The probability that a mosquito is infected at generation i (denoted σ imc where c is signifies the treatment arm) in the control group (that is, c =0) is described in equation (2): Assuming that the ATV acts to reduce the probability of transmission from mouse to mosquito, in the intervention group this probability is described in equation (3): where v is the effect size. This model is show diagrammatically in Supplementary Fig. S1 . A chain binomial model can then be constructed to calculate, given estimates of the three parameters r , s and v , the expected prevalence of infection in mice and mosquitoes at each generation is described in equation (4): Or more generally: Maximum likelihood estimation Let x i be the observed number of infected mice in generation i and n i the number of mice that were bitten. Similarly let y i be the observed number of infected mosquitoes in generation i and z i the number of mosquitoes that were fed. Using the notation to denote the corresponding list of observations, under a binomial model, the data likelihood is proportional to equation (5): This likelihood can be maximized to obtain estimates of r, s and v from the experimental data. Confidence intervals for the parameters were obtained from the profile likelihood. Spatial distribution of malaria transmission intensity The basic reproduction number for malaria, Pf R 0 , quantifies the potential for the disease to spread within a naive population [30] , [31] . The same metric for scenarios moderated by malaria control has been termed Pf R c ( [5] ). A full description of the data and methods used to generate a contemporary global map of estimated Pf R c for the year 2010 has been reported previously [26] . In brief, routine case reporting data (annual parasite incidence) for 13,449 administrative units in 43 endemic countries were sourced to define the spatial limits of P. falciparum transmission in 2010. A total of 22,212 P. falciparum parasite rate ( Pf PR) surveys were then used in a model-based geostatistical (MBG) prediction to create a continuous contemporary surface of malaria endemicity (the P. falciparum parasite rate, age-standardized to the 2–10 year age range, Pf PR 2–10 ) within these limits. A malaria transmission model was then utilized to describe the relationship between Pf PR and Pf R c . The model assumed that infections by different parasite types can accumulate in a single human host (super infection), and that they clear independently. The model also assumed that exposure risk is distributed unevenly in the population (heterogeneous biting) but is well-characterized and described by a one-parameter family of γ distributions. The model ignores acquired immunity and its effects, and the steady-state assumption implies that a population has been exposed for some time, so it is most suitable for describing malaria prevalence in older children, that is, for Pf PR 2–10 . This model was then used to convert the predicted values of Pf PR 2–10 at each pixel into equivalent predictions of Pf R c . In the present study, the resulting map was classified according to our target threshold of Pf R c values above or below 1.255. How to cite this article: Blagborough, A. M. et al . Transmission-blocking interventions eliminate malaria from laboratory populations. Nat. Commun. 4:1812 doi: 10.1038/ncomms2840 (2013).